Deciphering Fur transcriptional regulatory network highlights its complex role beyond iron metabolism inEscherichia coli The ferric uptake regulator (Fur) plays a critical role in the transcriptional regulation of iron metabolism. However, the full regulatory potential of Fur remains undefined. Here we comprehensively reconstruct the Fur transcriptional regulatory network in Escherichia coli K-12 MG1655 in response to iron availability using genome-wide measurements. Integrative data analysis reveals that a total of 81 genes in 42 transcription units are directly regulated by three different modes of Fur regulation, including apo - and holo -Fur activation and holo -Fur repression. We show that Fur connects iron transport and utilization enzymes with negative-feedback loop pairs for iron homeostasis. In addition, direct involvement of Fur in the regulation of DNA synthesis, energy metabolism and biofilm development is found. These results show how Fur exhibits a comprehensive regulatory role affecting many fundamental cellular processes linked to iron metabolism in order to coordinate the overall response of E. coli to iron availability. Iron is essential for many fundamental cellular processes, including N 2 fixation, DNA synthesis, the tricarboxylic acid (TCA) cycle and respiration [1] . Its function depends on its incorporation into proteins either as an isolated ion or in a more complex form such as iron-sulphur (FeS) clusters or a haeme group. Unfortunately, although iron is essential for most organisms, it can also be extremely toxic under oxic environments. Its ability to interact with superoxide and hydrogen peroxide can generate the highly reactive and damaging hydroxyl radical species by Fenton or Haber–Weiss reactions [2] . Thus, the amount of cellular free iron should be carefully managed to protect cells from iron-induced toxicity. In most Gram-negative bacteria, including Escherichia coli , ferric uptake regulator (Fur) regulates iron metabolism to precisely control cytoplasmic iron levels. Although classical Fur regulation involves the binding of Fur-Fe 2+ to the promoter region as a repressor, recent studies have demonstrated that Fur-Fe 2+ can function as an activator [3] , [4] and even Fur without an iron cofactor can act as both in some pathogenic bacteria [1] , [5] , [6] , [7] . In E. coli , the general role of Fur in iron metabolism has been extensively investigated from in vitro DNA-binding experiments and related mutation analysis [8] , [9] , [10] , [11] . However, much less is known about genome-scale in vivo Fur-binding events and the regulatory network they comprise. A complete reconstruction of the Fur transcriptional regulatory network in response to iron availability will reveal detailed modes of Fur regulation by emphasizing direct regulation and distinguishing them from indirect regulation. Furthermore, a better understanding of the Fur regulatory network can shed light on unanswered questions about its role in fundamental cellular processes, other than direct iron metabolism, that need to be coordinated when E. coli responds to iron availability. In this study, we apply a systems biology approach to decipher the Fur regulatory network in response to iron availability following the workflow shown in Fig. 1 . We integrate genome-scale data from chromatin immunoprecipitation (ChIP) with lambda exonuclease digestion followed by high-throughput sequencing (ChIP-exo) for Fur and RNA polymerase (RNAP) and from strand-specific massively parallel complementary DNA sequencing (RNA-seq). To fully reconstruct the Fur regulon, we examine the Fur-binding sites on the E. coli genome and if transcription at those sites is actively occurring based on RNAP-binding profiles. We also measure mRNA transcript levels on a genome scale to identify the direct Fur regulon. From this data, we then determine regulatory modes for individual open reading frames subject to Fur regulation and reported distinct mechanisms of apo - and holo -Fur activation (AA and HA) as well as holo -Fur repression (HR) in E. coli . Finally, we identify that the Fur regulatory network maintains intracellular iron concentration by connecting iron transport and utilization enzymes with negative/negative feedback loop pairs (−/−). The reconstruction of the Fur regulatory network provides a comprehensive view of the coordinative genome-wide regulatory role of this important global transcription factor (TF). 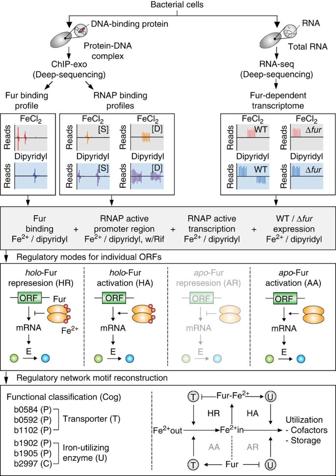Figure 1: Flowchart of the method. Thein vivogenome-wide Fur-binding maps, RNAP-binding profiles (S, static map; D, dynamic maps) and Fur-dependent transcriptomic data were generated under both iron-replete and iron starvation conditions. Combined data sets were used to determine direct Fur regulon and the regulatory mode for individual open reading frames (ORFs) governed by Fur. The Fur regulatory network was reconstructed by connecting iron transport and utilization regulatory motifs with negative-feedback loops. The regulatory modes (apo-Fur repression) and motifs (AA/AR pair) that are not identified in this study were presented in translucent format. Figure 1: Flowchart of the method. The in vivo genome-wide Fur-binding maps, RNAP-binding profiles (S, static map; D, dynamic maps) and Fur-dependent transcriptomic data were generated under both iron-replete and iron starvation conditions. Combined data sets were used to determine direct Fur regulon and the regulatory mode for individual open reading frames (ORFs) governed by Fur. The Fur regulatory network was reconstructed by connecting iron transport and utilization regulatory motifs with negative-feedback loops. The regulatory modes ( apo -Fur repression) and motifs (AA/AR pair) that are not identified in this study were presented in translucent format. Full size image Genome-wide identification of Fur-binding sites Previously, Fur-binding sites in E. coli have been characterized by in vitro DNA-binding experiments and related mutation analysis [8] , [11] ; however, direct measurement of in vivo Fur binding has not been available. We therefore first employed the ChIP-exo method to determine the in vivo Fur-binding maps with near 1-bp resolution in E. coli under both iron-replete (0.1 mM FeCl 2 ) and iron starvation (0.2 mM 2,2′-dipyridyl) [12] , [13] , [14] conditions ( Fig. 2a and Supplementary Fig. 1 ). In addition, we also examined active transcription sites on the E. coli genome by ChIP-exo analysis of RNAP under both static (with rifampicin that blocks transcription elongation) and dynamic (without rifampicin) conditions. 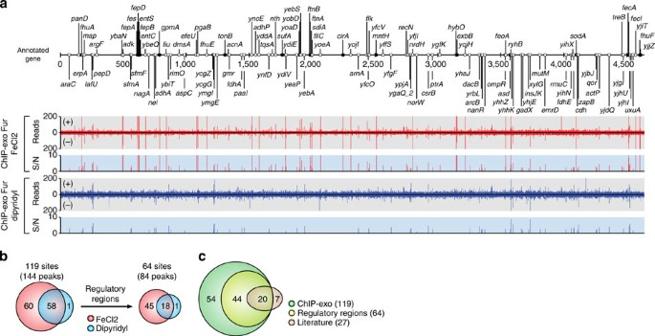Figure 2: Genome-wide distribution of Fur-binding sites. (a) An overview of Fur-binding profiles across theE. coligenome at mid-exponential growth phase under both iron-replete (red) and iron starvation (blue) conditions. Black and white dots indicate previously known and newly found Fur-binding sites, respectively. S/N denotes signal-to-noise ratio. (+) and (−) indicate forward and reverse reads, respectively. (b) Overlaps between Fur-binding sites under iron-replete and iron starvation conditions. (c) Comparison of the Fur-binding sites obtained from this study (ChIP-exo) with the literature information. Figure 2: Genome-wide distribution of Fur-binding sites. ( a ) An overview of Fur-binding profiles across the E. coli genome at mid-exponential growth phase under both iron-replete (red) and iron starvation (blue) conditions. Black and white dots indicate previously known and newly found Fur-binding sites, respectively. S/N denotes signal-to-noise ratio. (+) and (−) indicate forward and reverse reads, respectively. ( b ) Overlaps between Fur-binding sites under iron-replete and iron starvation conditions. ( c ) Comparison of the Fur-binding sites obtained from this study (ChIP-exo) with the literature information. Full size image Using a peak finding algorithm (MACE programme), 143 and 61 reproducible Fur-binding peaks were identified under iron-replete and iron starvation conditions, respectively ( Fig. 2a and Supplementary Data 1 ). The number of binding events was similar to those of other global TFs such as ArcA, Crp, Fnr and Lrp [15] , [16] , [17] , [18] . The high resolution of the ChIP-exo method enabled us to identify multiple binding peaks in several binding sites and separate binding peaks in divergent promoter regions ( Supplementary Fig. 2 ). In total, 118 and 59 Fur-binding sites where some sites contain multiple peaks were identified under iron-replete and iron starvation conditions, respectively. Most of the binding sites (58 of 59) under the iron starvation condition overlapped with those under the iron-replete condition, thus giving a total number of binding sites of 119 ( Fig. 2b ). One interesting exception was the upstream region of ycgZ - ymgA - ariR - ymgC , where Fur occupied only under the iron starvation condition, indicating possible direct regulation by Fur under this condition. Only 54% of binding sites (64 of 119) were located in putative regulatory regions (promoters and 5′-proximal to coding regions) and the remaining 46% were found in intragenic regions or between two coding regions of convergent genes. Based on RNAP-binding maps, we could confirm that bindings of Fur on the annotated non-regulatory regions were not related with active transcription events ( Supplementary Fig. 3 ). Before this study, 27 Fur-binding sites had been identified with strong experimental evidence [8] , [11] , 74% (20 of 27) of which were also detected in this study ( Fig. 2c and Supplementary Table 1 ). Collectively, a total of 98 Fur-binding sites were newly identified in this study, 45% (44 of 98) of which are located at putative regulatory regions ( Fig. 2c ), expanding the current scope of the Fur regulatory network. Genome-wide reconstruction of Fur regulon Currently, a total of 70 genes in 27 transcription units (TUs) have been characterized as members of Fur regulon to be directly regulated by Fur in E. coli based on strong experimental evidence [8] , [11] . From our ChIP-exo analysis, we significantly expanded the size of the potential Fur regulon to comprise 110 target genes in 64 TUs. To determine a causal relationship between Fur binding and transcript level, we compared transcript levels between wild-type and Δ fur mutant cells grown under both iron-replete and starvation conditions ( Supplementary Fig. 1 ). Overall, a total of 678 genes were differentially expressed with log2 fold change >0.5 and false discovery rate (FDR) <0.01 by the Fur deletion under either iron-replete (553) or iron starvation (211) conditions, 86 of which overlapped in both conditions ( Supplementary Fig. 4 and Supplementary Data 2 and 3 ). Combining our ChIP-exo results of Fur-binding maps with Fur-dependent transcriptome data, we could clarify target genes for direct Fur regulation depending on iron availability. A total of 81 genes in 42 TUs were directly regulated by Fur under either iron-replete (77 genes) or iron starvation (4 genes) conditions ( Fig. 3a,b and Supplementary Data 1 and Supplementary Table 2 ). These genes were placed into clusters of orthologous groups (COG) categories according to their functional annotation ( Fig. 3c ). As expected, the COG category for inorganic ion transport and metabolism (P) was found to be statistically overrepresented (hypergeometric P -value <0.05). In addition, two other categories for energy production and conversion (C) and secondary metabolites transport and metabolism (Q) were also overrepresented ( P -value <0.05). A diverse range of COG functional categories indicate that Fur may play complicated regulatory roles beyond iron metabolism to coordinate associated cellular processes. 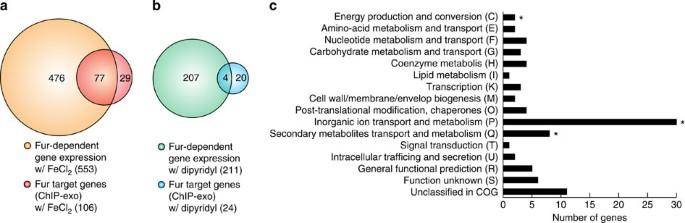Figure 3: Genome-wide identification of Fur regulon. Comparison of ChIP-exo results and gene expression profiles under (a) iron-replete and (b) iron starvation conditions to distinguish direct and indirect Fur regulon. (c) Functional classification of genes directly regulated by Fur. The asterisk indicates hypergeometricP-value <0.05. We also found that 30 of 81 genes in direct Fur regulon were regulated by 23 other TFs ( Supplementary Table 3 ). Interestingly, genes involved in suf system for the assembly of iron-sulphur clusters were regulated by additional five TFs (OxyR, NsrR, IscR, IhfB and IfhA) representing the importance of tight regulation of this operon depending on the various environmental changes. The remaining 51 genes were not regulated by other TFs, meaning that Fur exclusively regulates these genes in response to iron availability. Figure 3: Genome-wide identification of Fur regulon. Comparison of ChIP-exo results and gene expression profiles under ( a ) iron-replete and ( b ) iron starvation conditions to distinguish direct and indirect Fur regulon. ( c ) Functional classification of genes directly regulated by Fur. The asterisk indicates hypergeometric P -value <0.05. Full size image The 597 genes, which were Fur-dependent genes but not direct Fur regulon ( Fig. 3a,b ), would be targets for either indirect Fur regulation (mediated by RyhB small RNA), other iron-responsive TFs, or other stress-responsive TFs, as iron availability can generate different types of damage such as redox imbalance and oxidative stress [19] . As expected, none of the Fur-binding events within non-regulatory regions where we confirmed that active transcription was not occurring based on RNAP ChIP-exo data significantly changed the level of transcription of relevant target genes (log2 fold change <0.5 and FDR >0.01). Also, we found that 95% (55 of 58) of overlapped binding regions where Fur binds regardless of iron availability were not significantly related with the transcriptional regulation (log2 fold change <0.5 and FDR >0.01, Supplementary Data 1 ). Regulatory modes of Fur in response to iron availability An interesting aspect of the regulatory modes of Fur is its variable response to iron availability. Classical Fur regulation involves the binding of iron-bound Fur to the promoter region as a repressor; however, recent studies have shown cases where Fur functions as an activator [3] , [4] or as both even in the absence of its iron cofactor in some pathogenic species [1] , [5] , [6] . In order to define regulatory modes of Fur in E. coli , we classified the regulation of 81 genes that are directly regulated by Fur into three different modes (HR, HA and apo -Fur activation) depending on changes in transcript levels and Fur binding with/without iron. For example, the promoter regions of fepA and fes TUs, where two divergent promoters exist, were extensively occupied by Fur under the iron-replete condition and this binding significantly decreased transcript levels under this condition ( Fig. 4a , HR). We denoted this regulatory mode as HR. A total of 65 genes were regulated by this mode, and 23 of them were previously investigated with either weak evidence such as comparative transcriptomic analysis ( fiu-ybiX , efeUOB , fhuE , yncE , yddA-yddB , ydiE , nrdHIEF , yqjH and feoABC ) or no evidence ( ybaN , adhP , ynfD , yoeA and yojI ; Supplementary Data 1 ). Interestingly, the efeUOB operon, which encodes a ferrous iron transporter complex, was found to be still repressed by iron-bound Fur, even though this operon is cryptic due to a frameshift mutation [20] . The calculation of relative distance from Fur bindings to transcription start site (TSS) [8] , [11] , [21] showed that Fur bindings are localized to around the RNAP-binding regions ( Supplementary Fig. 5a and Supplementary Data 1 ). As is already known, the direct repression of transcription by Fur seems to be achieved by exclusion of RNAP binding because of the occupancy of Fur at this region. 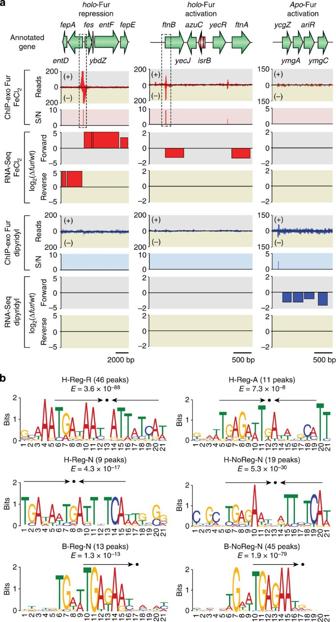Figure 4: Regulatory modes of individual open reading frames governed by Fur in response to iron availability. (a) Examples ofholo-Fur repression (HR) mode (fepA-entDandfes-ybdZ-entF-fepE),holo-Fur activation (HA) mode (ftnBandftnA) andapo-Fur activation (AA) mode (ycgZ-ymgA-ariR-ymgC). S/N denotes signal-to-noise ratio. (+) and (−) in ChIP-exo data indicate forward and reverse reads, respectively. Boxes with dotted lines are zoom-in examples inSupplementary Fig. 2. (b) Sequence logo representations of the Fur-DNA-binding profiles with consensus sequence highlighted with arrows. H-Reg-R,holo-Fur repression; H-Reg-A,holo-Fur activation; H-Reg-N,holo-Fur-binding peaks in regulatory regions but no change in transcript level; H-NoReg-N,holo-Fur-binding peaks in non-regulatory regions; B-Reg-N, binding peaks regardless of iron availability in regulatory regions but no change in transcript; B-NoReg-N, binding peaks regardless of iron availability in non-regulatory regions. Figure 4: Regulatory modes of individual open reading frames governed by Fur in response to iron availability. ( a ) Examples of holo -Fur repression (HR) mode ( fepA-entD and fes-ybdZ-entF-fepE ), holo -Fur activation (HA) mode ( ftnB and ftnA ) and apo -Fur activation (AA) mode ( ycgZ-ymgA-ariR-ymgC ). S/N denotes signal-to-noise ratio. (+) and (−) in ChIP-exo data indicate forward and reverse reads, respectively. Boxes with dotted lines are zoom-in examples in Supplementary Fig. 2 . ( b ) Sequence logo representations of the Fur-DNA-binding profiles with consensus sequence highlighted with arrows. H-Reg-R, holo -Fur repression; H-Reg-A, holo -Fur activation; H-Reg-N, holo -Fur-binding peaks in regulatory regions but no change in transcript level; H-NoReg-N, holo -Fur-binding peaks in non-regulatory regions; B-Reg-N, binding peaks regardless of iron availability in regulatory regions but no change in transcript; B-NoReg-N, binding peaks regardless of iron availability in non-regulatory regions. Full size image In contrast, associations of Fur on the ftnB and ftnA TUs increased transcript levels under the iron-replete condition ( Fig. 4a , HA). Thus, we denoted this regulatory mode as HA. In the previous study, only ftnA was thought to be a direct target for activation by Fur binding at the region upstream of the promoter to prevent binding of other repressors [4] . However, we identified 11 more target genes ( argF-yagI , adk , ftnB , hybOA , zapB , uxuAB , acnA and yjiT ) for direct activation by iron-bound Fur ( Supplementary Data 1 ). Most of them utilize iron ( ftnB , hybOA , uxuA and acnA ) or other divalent metal ions ( argF , adk and uxuB ) as cofactors or activators. Although acnA -encoding aconitase that catalyse the inter-conversion of citrate and isocitrate in TCA cycle and sense iron starvation and oxidative stress was known to be indirectly regulated by Fur via RyhB-mediated mRNA degradation [10] , it was also directly activated by iron-bound Fur. This observation is in agreement with the northern blot analysis from the previous study where Δ ryhB Δ fur double mutant showed much less amounts of acnA transcript compared with the Δ ryhB mutant, presumably due to the loss of direct activation by Fur [10] . In this case, Fur binds to the sites either further upstream or downstream of the promoter region, unlike HR sites, where Fur binds to the RNAP-binding regions ( Supplementary Fig. 5b and Supplementary Data 1 ). This suggests that Fur may prevent binding of other repressors like in the case of ftnA [4] or directly activate transcription through additional mechanisms such as recruiting RNAP [3] , [22] to activate transcription. Another aspect of Fur is its regulation mediated by binding of its iron-free form in some pathogenic bacterial species [1] , [5] , [6] . Although E. coli K-12 MG1655 has been considered to not have this regulatory mode, we observed that the promoter region of the ycgZ-ymgA-ariR-ymgC operon is bound by Fur only under the iron starvation condition, and this binding was accompanied with an increase in transcript level ( Fig. 4a , apo -Fur activation). We denoted this regulatory mode as apo -Fur activation (AA). Based on the distance calculation from Fur binding to TSS (−74 relative to TSS), we believe that apo -Fur activation of this operon might also occur by either preventing binding of other repressors or directly recruiting RNAP ( Supplementary Data 1 ). Three genes ( ymgA , ariR and ymgC ) in this operon are associated with biofilm formation and one of them ( ariR ) is also related to acid resistance [23] . Thus, Fur could play a key role in the suppression of biofilm formation and resistance to acidic stress by activating this particular operon under the iron starvation condition. We did not observe the regulatory mode of apo -Fur repression (AR) for any TU in E. coli K-12 MG1655, although some pathogenic strains have been reported to have this mode [1] , [5] , [6] . To further analyse the sequences of individual Fur-binding sites, we created six different data sets with footprint sequences based on Fur-binding modes (with or without iron), binding locations (regulatory or non-regulatory region) and change of transcript level (repression, activation or no change in transcript level) as follows: 46 binding peaks in HR (H-Reg-R), 11 binding peaks in HA (H-Reg-A), 9 holo -Fur-binding peaks in regulatory regions but no change in transcript level (H-Reg-N), 19 holo -Fur-binding peaks in non-regulatory regions (H-NoReg-N), 13 binding peaks regardless of iron availability in regulatory regions but no change in transcript (B-Reg-N) and 45 binding peaks regardless of iron availability in non-regulatory regions (B-NoReg-N). We also arbitrarily extended the sequence of each site by 20 nt at each end to allow for adjacent sequences to be included in the motif search procedure [24] . The motif search for holo -Fur-repressed genes yielded a consensus sequence ( TRAKAAYSATTATYA ) with canonical Fur boxes containing an internal palindromic 7-1-7 sequence ( TGATAATnATTATCA ) [25] ( Fig. 4b , H-Reg-R). In contrast, the identified motifs for holo -Fur-activated genes ( TGAGAWTGATWHKCM ; Fig. 4b , H-Reg-A), holo -Fur-binding sites in regulatory regions without transcript level change ( TGADAWTGATTHTCA ; Fig. 4b , H-Reg-N) and those in non-regulatory regions ( YGAKAWYVDTTMTCA ; Fig. 4b , H-NoReg-N) were also similar to previously identified Fur boxes but had a relatively weak palindromic sequence with sequence diversity as revealed in the ftnA study [4] . Interestingly, the other two cases where Fur binds regardless of iron availability to either regulatory ( TGAKARY ; Fig. 4b , B-Reg-N) or non-regulatory ( TGAGAAT ; Fig. 4b , B-NoReg-N) regions resembled just the half of the previously known Fur boxes. A consensus sequence for AA mode was not identified because it only had one binding peak. As the known apo -Fur-binding motif ( AATGA ) was only specific for AR and not for apo -Fur activation in Helicobacter pylori [5] , we also could not find the similar motif in the region of apo -Fur binding that stimulates expression ( Supplementary Table 4 ). As genome-wide TF binding data from ChIP experiments can be a source of information for inferring the relative DNA-binding affinity of this protein in vivo [26] , we assigned a signal-to-noise (S/N) ratio of each Fur-binding peak to in vivo relative binding affinity of each site ( Supplementary Data 1 ). The more the binding sequence differed from the consensus Fur box, the lower the in vivo relative binding affinity became ( R 2 =0.52; Supplementary Fig. 6 ). The holo -repressed genes (H-Reg-R) showed significantly higher in vivo relative binding affinity compared with other holo -Fur bindings (H-Reg-A, H-Reg-N and H-NoReg-N) as well as non-specific Fur bindings (B-Reg-N and B-NoReg-N; Supplementary Fig. 7 ; Wilcoxon rank-sum test, P <0.01). However, the in vivo relative binding affinity of H-Reg-A sites were similar to those of H-Reg-N and H-NoReg-N sites, indicating that binding affinity alone cannot be the single determinant as to whether regulation occurs or not [27] . Also, two non-specific binding sites (B-Reg-N and B-NoReg-N) showed significantly lower relative binding affinity than the other four holo -Fur-binding categories, presumably due to the presence of only half of the consensus motif in these sites ( Supplementary Fig. 7 ; Wilcoxon rank-sum test, P <0.01). Given these binding properties of Fur, it is plausible that there might be additional undiscovered functions for Fur, or evolution has been slow to eliminate these non-specific interactions with low affinity (half of consensus motif) for Fur as shown in other cases [15] , [16] , [27] , [28] . Fur-regulated feedback loop motifs for iron metabolism Next, we reconstructed the Fur regulatory network in E. coli to observe how Fur regulates genes for iron metabolism. After the functional classification of 81 genes directly regulated by Fur, we observed that the functions of 53% (43 genes) of those genes were mainly localized to iron transport and metabolism. To identify the metabolic pathways regulated by Fur, the members of Fur regulon were mapped to the iron uptake/utilization pathways [2] , [8] , [9] , [29] ( Fig. 5a ). Under the iron-replete condition, Fur repressed entire enterobactin biosynthesis/transport and iron or iron-complex transport systems including fhuE , feoABC and fiu . On the other hand, it activated several iron-utilizing enzymes including ftnB , uxuAB and hybOA under the same condition. As shown in a previous study, one of the FeS cluster assembly systems mediated by suf operon is directly regulated by Fur, whereas the other mediated by the isc operon is indirectly regulated by Fur via RyhB-mediated mRNA degradation [30] . This RyhB-mediated regulation also forces genes associated with iron utilization to be regulated according to the intracellular iron pool ( sdhDC , fumA , bfr ). 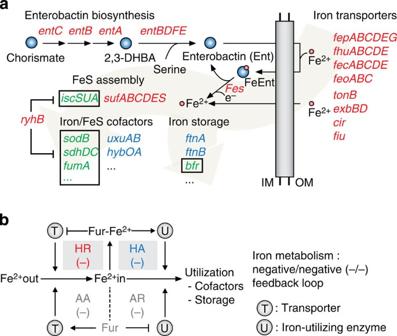Figure 5: Iron acquisition/utilization pathways directly regulated by Fur and regulatory network motif. (a) The iron acquisition (enterobactin biosynthesis and iron/enterobatin transport), iron utilization (iron storage and iron/FeS cofactors) and FeS assembly pathways are represented. The genes regulated by HR and HA are depicted by red and blue characters, respectively. The genes regulated by RyhB-mediated mRNA degradation are depicted by green characters with black boxes. 2,3-DHBA, 2,3-dihydroxybenzoic acid; IM, inner membrane; OM, outer membrane. (b) Schematic diagram for the Fur regulatory motif reconstruction for iron metabolism. Shaded grey boxes indicate motif loops utilized byE. coliK-12 MG1655 for iron metabolism (negative/negative feedback loop motifs achieved by HR/HA modes of regulation). Figure 5: Iron acquisition/utilization pathways directly regulated by Fur and regulatory network motif. ( a ) The iron acquisition (enterobactin biosynthesis and iron/enterobatin transport), iron utilization (iron storage and iron/FeS cofactors) and FeS assembly pathways are represented. The genes regulated by HR and HA are depicted by red and blue characters, respectively. The genes regulated by RyhB-mediated mRNA degradation are depicted by green characters with black boxes. 2,3-DHBA, 2,3-dihydroxybenzoic acid; IM, inner membrane; OM, outer membrane. ( b ) Schematic diagram for the Fur regulatory motif reconstruction for iron metabolism. Shaded grey boxes indicate motif loops utilized by E. coli K-12 MG1655 for iron metabolism (negative/negative feedback loop motifs achieved by HR/HA modes of regulation). Full size image From this analysis, we were able to connect transport and utilization feedback loop pairs [31] ( Fig. 5b ). In the left loop, Fur regulates transcription of the transport protein (T) in either the presence or the absence of iron, facilitating the uptake of the iron (Fe 2+ out ), whereas in the right loop, Fur controls transcription of iron-utilization enzymes (U) that store Fe 2+ in or use it as cofactors. The possible logical structures of the feedback loop motifs can be characterized depending on how Fur-Fe 2+ (or Fur) represses or activates both T and U. In our case, the Fur regulatory network showed negative/negative motif loop pairs (−/−) for iron metabolism to maintain intracellular iron concentration by repressing the transcription of iron transporter genes (HR) and enhancing the production of iron-utilizing proteins (HA) under the iron-replete condition ( Fig. 5b ). Based on this rule, we suggest that the function of nine Y-genes ( yncE , yddA-yddB , ydiE , yqjH , ybaN , ynfD , yoeA and yojI ) directly regulated by HR mode might be involved in either iron/iron-complex transportation or iron-acquisition processes given their putative functional annotations as transporters or membrane proteins [8] , [9] . In addition, there is growing evidence that Fur in pathogenic species also have an AA mode for iron transporters and an AR mode for iron utilization enzymes ( Supplementary Table 5 ). Because the other negative/negative motif loop pair (−/−) can also be achieved by regulating target genes under AA and AR modes ( Fig. 5b ), these pathogenic species might have evolved to have additional iron acquisition/utilization regulatory systems in order to more sensitively respond to iron availability. The comprehensive genome-scale reconstruction of the Fur regulatory network in E. coli provided us with strong evidence to extend the scope of its direct roles in response to iron availability other than iron uptake and utilization ( Fig. 6a ). First, although Fur is known to be involved in the regulation of the nrdHIEF operon encoding the Mn 2+ -dependent ribonucleotide reductase system (Mn-RNR) without direct Fur-binding evidence [32] , we found that Fur actually binds to the upstream region of the nrdHIEF operon and directly regulated their expression to provide dexoyribonucleotide precursors for DNA synthesis using Mn 2+ under the iron starvation condition ( Fig. 6b ). We believe the regulation of mntH , which encodes divalent metal cation transporter (preferentially Mn 2+ ) by Fur, would help this process. Second, Fur also directly activated one of the TCA enzymes encoded by acnA under the iron-replete condition in addition to indirect repression of it by RyhB under the iron starvation condition ( Fig. 6c ) [10] . This dual regulation of acnA by Fur might enable cells to rapidly change flux of the TCA cycle between fermentative pathways and oxidative phosphorylation in response to iron availability, which is in agreement with the prediction of the genome-scale model of metabolism and gene expression (ME-Model) of E. coli [33] ( Supplementary Fig. 8 ) as well as experimental results in the previous study using Staphylococcus aureus [34] . Finally, we found that the apo -Fur activation of ymgA , ymgC and ariR would suppress biofilm formation in addition to apo -IscR regulation [35] and enable planktonic growth of the cells to find an iron-rich environment [23] ( Fig. 6d ). Also, activation of ariR would contribute to expressing genes to endure acidic environments caused by shifting the metabolic state towards fermentative pathways under the iron starvation condition. 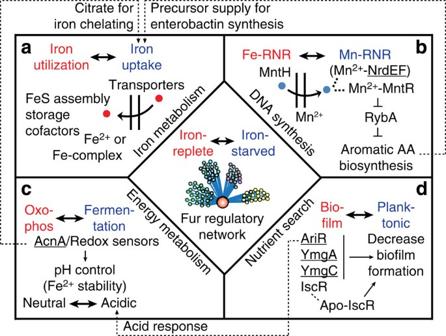Figure 6: Global coordination roles of the Fur regulatory network inE. coli. The Fur regulatory network is involved in many cellular functions required in addition to iron acquisition and utilization. Fur directly regulates genes associated with (a) iron metabolism, (b) DNA synthesis, (c) redirection of metabolism towards fermentative pathways and (d) biofilm formation for searching nutrients in response to iron availability. These networks are linked through the coordination role that Fur plays. Underlined characters indicate novel Fur regulon revealed in this study. Figure 6: Global coordination roles of the Fur regulatory network in E. coli . The Fur regulatory network is involved in many cellular functions required in addition to iron acquisition and utilization. Fur directly regulates genes associated with ( a ) iron metabolism, ( b ) DNA synthesis, ( c ) redirection of metabolism towards fermentative pathways and ( d ) biofilm formation for searching nutrients in response to iron availability. These networks are linked through the coordination role that Fur plays. Underlined characters indicate novel Fur regulon revealed in this study. Full size image Remarkably, these networks were connected to each other. For example, Mn 2+ uptake and temporal TCA shutdown, driven by Fur under iron starvation condition, consequently led to an increase in the intracellular Fe 2+ pool [36] , and Fur-mediated repression of biofilm formation contributes to protecting cells from acidic environments caused by temporal TCA shutdown under this condition. Thus, disrupting the Fur regulatory network in either iron-replete or iron starvation conditions can lead to dramatic changes in transcript levels of genes. Besides Fur direct regulon, these genes can be associated with other iron-responsive TFs or various stress responses, including oxidative stress, redox imbalance and acidic environment ( Supplementary Tables 6 and 7 ). This could be the reason why only a small fraction of the Fur-dependent genes was directly regulated by Fur in this study (81 of 678) as in other studies [37] , [38] . The Fur regulon has been studied recently on a genome scale in a variety of proteobacteria: Caulobacter crescentus (α-proteobacteria) [39] , Geobacter sulfurreducens (δ-proteobacteria) [37] , Vibrio cholerae (γ-proteobacteria) [40] and Campylobacter jejuni (ɛ-proteobacteria) [6] . We investigated how E. coli Fur and its direct regulon (81 genes) have been evolved and regulated in proteobacteria phylum by comparing E. coli with other six proteobacteria including those four species, Klebsiella pneumonia (γ-proteobacteria) and Ralstonia solanacearum (β-proteobacteria). We first compared the homology of Fur in E. coli K-12 MG1655 with those in other species ( Supplementary Fig. 9 ). As expected, Fur was highly conserved in γ-proteobacteria, but relatively less conserved in other classes of proteobacteria. Interestingly, the ratio of Fur-regulated orthologues to the known Fur regulon in each species was correlated with the degree of conservation of Fur ( Supplementary Fig. 10 and Supplementary Table 8 ). These results indicate that Fur might have evolved to have diverse roles in other proteobacteria by regulating different biological processes or adding additional layers of regulation using small RNAs (sRNAs) or TFs: V. cholera Fur regulates ribosome formation and several unique sRNAs [40] ; C. crescentus Fur regulates riboflavin biosynthesis and additional TFs [39] ; G. sulfurreducens Fur extensively regulates central metabolism primarily associated with the TCA cycle and additional iron-responsive TF (IdeR) but no sRNAs [37] . In summary, we have described an integrative analysis of various types of genome-scale experimental data and how this systems approach enabled us to comprehensively understand the complex roles of the Fur regulatory network in E. coli . By combining ChIP-exo, which showed higher resolution and lower false-discovery rates than conventional ChIP-chip or ChIP-seq [27] , with highly sensitive RNA-seq-based transcriptome analysis [41] , we showed an unprecedented view into genome-wide binding of E. coli Fur and its regulon as well as its complex regulatory network. In the future, the incorporation of these comprehensive operon structures that account for cellular regulation along with regulatory networks [42] into ME-Model would make it possible to mechanistically model and predict the complex regulatory interactions and thus allow us to more accurately compute complex phenotypes [43] . Bacterial strains, primers, media and growth conditions All strains used are E. coli K-12 MG1655 and its derivatives. The E. coli strain harbouring Fur-8myc was generated by a λ Red-mediated site-specific recombination system targeting C-terminal region of fur and confirmed by western blot analysis ( Supplementary Fig. 11 ) [44] . Deletion mutant (Δ fur ) was also constructed by a λ Red-mediated site-specific recombination system [45] . Glycerol stocks of E. coli strains were inoculated into M9 minimal medium (47.8 mM Na 2 HPO 4 , 22 mM KH 2 PO 4 , 8.6 mM NaCl, 18.7 mM NH 4 Cl, 2 mM MgSO 4 and 0.1 mM CaCl 2 ) supplemented with 0.2% (w/v) glucose and cultured overnight at 37 °C with vigorous agitation. For the iron-replete condition, the overnight cultures were inoculated into the same fresh M9 medium with 0.1 mM FeCl 2 and continued to culture at 37 °C with vigorous agitation to mid-log phase. For the iron starvation condition, the overnight cultures inoculated into the same fresh M9 media were supplemented with 0.2 mM 2,2′-dipyridyl at early-log phase and continued to culture at 37 °C for additional 2 h with vigorous agitation ( Supplementary Fig. 1 ). For the rifampicin-treated cultures, the rifampicin dissolved in methanol was added to a final concentration of 150 μg ml −1 at mid-log phase and stirred for 20 min. ChIP-exo To identify Fur- and RNAP-binding maps in vivo , we isolated the DNA bound to Fur protein and RNAP from formaldehyde crosslinked E. coli cells by ChIP with the specific antibodies (1:50 dilution) that specifically recognizes myc tag (9E10, Santa Cruz Biotechnology) and RpoB subunit of RNAP (NT63, Neoclone), respectively, and Dynabeads Pan Mouse IgG magnetic beads (Invitrogen) followed by stringent washings as described previously [16] . ChIP materials (chromatin-beads) were used to perform on-bead enzymatic reactions of the ChIP-exo method [46] with following modifications. Briefly, the sheared DNA of chromatin beads was repaired by the NEBNext End Repair Module (New England Biolabs) followed by the addition of a single dA overhang and ligation of the first adaptor (5′-phosphorylated) using dA-Tailing Module (New England Biolabs) and NEBNext Quick Ligation Module (New England Biolabs), respectively. Nick repair was performed by using PreCR Repair Mix (New England Biolabs). Lambda exonuclease- and RecJ f exonuclease-treated chromatin was eluted from the beads and the protein–DNA crosslink was reversed by overnight incubation at 65 °C. RNAs- and Proteins-removed DNA samples were used to perform primer extension and second adaptor ligation with following modifications. The DNA samples incubated for primer extension as described previously [46] were treated with dA-Tailing Module (New England Biolabs) and NEBNext Quick Ligation Module (New England Biolabs) for second adaptor ligation. The DNA sample purified by GeneRead Size Selection Kit (Qiagen) was enriched by PCR using Phusion High-Fidelity DNA Polymerase (New England Biolabs). The amplified DNA samples were purified again by GeneRead Size Selection Kit (Qiagen) and quantified using Qubit dsDNA HS Assay Kit (Life Technologies). Quality of the DNA sample was checked by running Agilent High Sensitivity DNA Kit using Agilent 2100 Bioanalyzer (Agilent) before sequenced using MiSeq (Illumina) in accordance with the manufacturer’s instructions. Each modified step was also performed in accordance with the manufacturer’s instructions. ChIP-exo experiments were performed in biological duplicate. RNA-seq expression profiling Total RNA including small RNAs was isolated using the cells treated with RNAprotect Bacteria Reagent (Qiagen) followed by purification using Qiagen RNeasy Plus Mini Kit (Qiagen) in accordance with the manufacturer’s instruction. Samples were then quantified using a NanoDrop 1000 spectrophotometer (Thermo Scientific) and quality of the isolated RNA was checked by running RNA 6000 Pico Kit using Agilent 2100 Bioanalyzer (Agilent). Paired-end, strand-specific RNA-seq was performed using the dUTP method [41] with the following modifications. The ribosomal RNAs were removed with Ribo-Zero rRNA Removal Kit (Epicentre). Subtracted RNA was fragmented for 2.5 min using RNA Fragmentation Reagents (Ambion). Complementary DNA was generated using SuperScript III First-Strand Synthesis protocol (Invitrogen) with random hexamer priming. The samples were sequenced using MiSeq (Illumina) in accordance with the manufacturer’s instructions. RNA-seq experiments were performed in biological duplicate. ChIP-exo output processing Sequence reads generated from ChIP-exo were mapped onto the reference genome (NC_000913.2) using bowtie [47] with default options to generate SAM output files. MACE programme ( https://code.google.com/p/chip-exo/ ) was used to define peak candidates from biological duplicates for each experimental condition with sequence depth normalization. To reduce false-positive peaks, peaks with S/N ratio less than 1.5 were removed. The noise level was set to the top 5% of signals at genomic positions because top 5% resembles background level in plateau ( Supplementary Fig. 12a ) and top 5% intensities from each ChIP-exo replicates across conditions correlate well with the total number of reads ( Supplementary Fig. 12b ). The calculation of S/N ratio resembles the way to calculate ChIP-chip peak intensity where IP signal was divided by Mock signal [15] , [16] . Then, each peak was assigned to the nearest gene. Genome-scale data were visualized using MetaScope ( http://systemsbiology.ucsd.edu/Downloads/MetaScope ) and NimbleGen’s SignalMap software. Motif search and analysis The Fur-binding motif analysis was completed using the MEME tool from the MEME software suite [48] . We extended the sequence of each binding site by 20 bp at each end to allow for adjacent sequences to be included in the analysis. We used default settings except for the width parameter fixed at 21 bp. Potential motifs for each case were further processed with FIMO ( P <0.0001) [48] . FIMO results were filtered by using the regions around the ChIP-exo-binding sites (100 bp extended at each end of binding sites) to obtain a map of all motifs. RNA-seq output processing Sequence reads generated from RNA-seq were mapped onto the reference genome (NC_000913.2) using bowtie [47] with the maximum insert size of 1,000 bp, and two maximum mismatches after trimming 3 bp at 3′ ends. SAM files from bowtie, then, were used for Cufflinks ( http://cufflinks.cbcb.umd.edu/ ) [49] and Cuffdiff to calculate fragments per kilobase of exon per million fragments (FPKM) and differential expression, respectively. Cufflinks and Cuffdiff were run with default options with library type of dUTP RNA-seq with default normalization method (classic-fpkm). From cuffdiff output, genes with differential expression with log2 fold change >0.5 and a FDR value <0.01 were considered as differentially expressed genes. Genome-scale data were visualized using MetaScope ( http://systemsbiology.ucsd.edu/Downloads/MetaScope ) and NimbleGen’s SignalMap software. COG functional enrichment Direct Fur regulons were categorized according to their annotated COG category. Functional enrichment of COG categories in Fur-regulated genes was determined by performing one-tailed Fisher’s exact test (Hypergeometric test), and P -value <0.05 was considered significant. Three categories (energy production and conversion, inorganic ion transport and metabolism, and secondary metabolites transport and metabolism) were statistically overrepresented. Conservation analysis of Fur regulon Gene annotation of six other strains, Vibrio, Geobacter, Caulobacter, Campylobacter, Klebsiella and Ralstonia, were obtained from the SEED server ( http://theseed.org ) and orthologue calculation to E. coli K-12 MG1655 was also performed on RAST (Rapid Annotation using Subsystem Technology) server [50] . From RAST output, orthologous genes with bi-directional hits were only retained. Conservation level of fur and genes in Fur regulon were calculated from orthologue retained from RAST output. Western blot analysis Soluble cell lysates were subjected to electrophoresis in a NuPAGE Novex 10% Bis-Tris Gel (Invitrogen) with MOPS running buffer, and the resolved proteins were transferred to a Hybond-ECL membrane (Amersham Biosciences) using XCell II Blot Module (Invitrogen). The ECL Western detection kit (Amersham Biosciences), antibodies that specifically recognizes myc tag (9E10, Santa Cruz Biotechnology) and RpoB subunit of RNAP (NT63, Neoclone), respectively, and horseradish peroxidase (HRP)-conjugated sheep anti-mouse immunoglobulin G (IgG) (Amersham Biosciences) were used to detect the proteins. All antibodies were diluted with 1:10,000 ratio. The Qubit Protein Assay Kit (Invitrogen) was used to measure the amount of total proteins in the lysates in order to load the same amount of proteins in each lane. All experiments were performed in accordance with the manufacturer’s instructions. How to cite this article: Seo, S. W. et al . Deciphering Fur transcriptional regulatory network highlights its complex role beyond iron metabolism in Escherichia coli . Nat. Commun. 5:4910 doi: 10.1038/ncomms5910 (2014). Accession codes: All raw data for ChIP-exo and RNA-seq have been deposited in the Gene Expression Omnibus under the accession code GSE54901 .